Focused plasmonic trapping of metallic particles Scattering forces in focused light beams push away metallic particles. Thus, trapping metallic particles with conventional optical tweezers, especially those of Mie particle size, is difficult. Here we investigate a mechanism by which metallic particles are attracted and trapped by plasmonic tweezers when surface plasmons are excited and focused by a radially polarized beam in a high-numerical-aperture microscopic configuration. This contrasts the repulsion exerted in optical tweezers with the same configuration. We believe that different types of forces exerted on particles are responsible for this contrary trapping behaviour. Further, trapping with plasmonic tweezers is found not to be due to a gradient force balancing an opposing scattering force but results from the sum of both gradient and scattering forces acting in the same direction established by the strong coupling between the metallic particle and the highly focused plasmonic field. Theoretical analysis and simulations yield good agreement with experimental results. Research on metallic particles has attracted increasing attention owing to their special chemical and physical properties and extensive applications in various areas including biotechnology, catalysis, surface-enhanced Raman scattering and microfabrication [1] , [2] , [3] , [4] . This strongly motivates development of trapping and manipulation technologies for metallic particles. Optical tweezers, one of the contenders of trapping technologies, has naturally become a first choice because of its tremendous success in trapping dielectric particles. Trapping occurs when the attractive force (also called gradient force) because of intensity inhomogeneity overcomes the repulsive force (also called radiation pressure or scattering force) due to scattering and absorption of particles [5] , [6] , [7] . However, optical tweezers are not always successful in trapping large metallic particles. For Rayleigh metallic particles (with radius a << λ 0 , where λ 0 denotes the incident wavelength), stable trapping using optical tweezers is possible for particle diameters from 18 to 254 nm (ref. 8 ), where scattering forces are small because of deep-subwavelength particle sizes, and thus easily overcome by gradient forces [8] , [9] , [10] . In contrast, optical tweezers usually push metallic mesoscopic particles ( a ~ λ 0 ) and Mie particles ( a ≫ λ 0 ) away from the light spot because scattering forces strengthen more rapidly than gradient forces [7] . Although several special optical tweezers rely on the scattering force to confine Mie metallic particles in a ring-shaped potential well [11] , [12] , [13] , [14] , in practice these techniques suffer drawbacks, such as high-precision requirements in shaping and adjusting the laser beams and narrow-trapping regions. Thus, trapping metallic particles of different sizes using a simple universal method remains a significant challenge. In recent years, plasmonic tweezers, based on surface plasmon polaritons (SPPs) excited in metallic nanostructures, have exhibited an enhanced attractive force for both dielectric and metallic particles [15] , [16] , [17] , [18] , [19] , [20] , [21] , [22] , providing a potential means for trapping and manipulating metallic particles. In this article, we report a variant of the plasmonic tweezers for trapping and manipulating metallic particles that is based on a highly focused plasmonic field on a flat metal film excited by a radially polarized (RP) beam (also called plasmonic virtual probe [23] , [24] , [25] ). This variant can attract and trap both Rayleigh- and Mie-type metallic particles. In particular, trapping of mesoscopic/Mie particles is particularly successful. In experiments to support our claim, we choose metallic particles of diameters in the range 0.5–2.2 μm that require greater gradient forces to attain an equilibrium of forces than those for Rayleigh particles. In contrast, trapping failed when using focused optical tweezers in an identical experimental configuration but with the metal film removed. Through numerical analysis based on a three-dimensional (3D) finite difference time domain (FDTD) calculation and Maxwell stress tensor (MST) method, we find that the resultant total force in the optical tweezers is composed of weakly attracting gradient forces and a stronger repulsive scattering force, which is confirmed by experimental observations. Contrary to common assumptions, we find that the resultant total force in the plasmonic tweezers is the result not of a stronger gradient force dominating an opposing scattering force but instead of a dominant gradient force assisted by a weak scattering force acting in the same direction. The dominant gradient force originates from the coupling between a greatly enhanced SPP field and metallic particles, whereas the unusual scattering force is due to pushes exerted through focused SPP propagation. To the best of our knowledge, the experiments described here represent the first demonstration of plasmonic trapping of metallic particles with diameters above 500 nm. Thus, our plasmonic tweezers are not only capable of trapping metallic Rayleigh particles, but also show potential in trapping and manipulating larger metallic objects, such as nanowires or even complex micrometre-sized metallic structures. Compared with other plasmonic tweezers based on metallic microdisks or bowtie structures [20] , [21] , [22] , our set-up benefits from the structureless excitation of SPPs in a dynamic configuration, thereby reducing the need to fabricate nanometre-sized complex structures. Comparison of plasmonic and optical tweezers experiments The schematic of the plasmonic tweezers in Fig. 1a depicts a RP cylindrical vector beam focused by a high-numerical-aperture objective lens into a Kretschmann coupling-type glass plate top-coated with a thin gold film where SPPs are excited and form a sharp plasmonic virtual probe. The theoretical full width at half maximum of virtual probe is 261 nm (~0.245 λ 0 , λ 0 =1,064 nm is the incident wavelength) and the wavelength of excited SPPs is 754 nm. Gold particles diffused in water and injected into an in-house-fabricated chamber onto a gold film are manipulated by the plasmonic virtual probe. Detailed experimental set-up is presented in Fig. 1b and described in the Methods section. 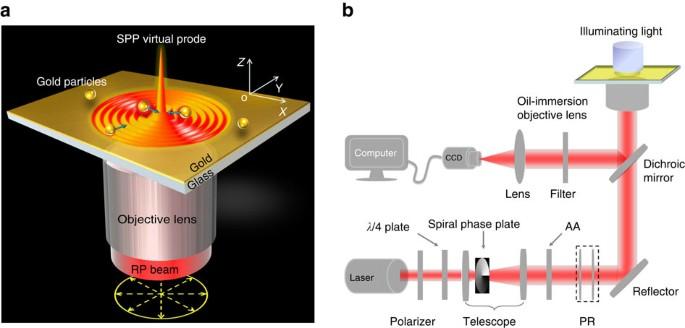Figure 1: Schematic diagram of experimental set-up. (a) Schematic of trapping metallic particles by a SPP virtual probe. Bottom yellow arrows indicate the polarized directions of the RP beam; blue arrows indicate the direction of force on each gold particle in the SPP virtual probe field. (b) Experimental set-up of the focused plasmonic trapping system. The incident wavelength isλ0=1,064 nm, the thickness of the thin gold film is 45 nm, the refractive index of the glass substrate is 1.515, the diameter of the gold particles is 1±0.1 μm. The theoretical full width at half maximum of the SPP virtual probe is 261 nm (~0.245λ0). Figure 1: Schematic diagram of experimental set-up. ( a ) Schematic of trapping metallic particles by a SPP virtual probe. Bottom yellow arrows indicate the polarized directions of the RP beam; blue arrows indicate the direction of force on each gold particle in the SPP virtual probe field. ( b ) Experimental set-up of the focused plasmonic trapping system. The incident wavelength is λ 0 =1,064 nm, the thickness of the thin gold film is 45 nm, the refractive index of the glass substrate is 1.515, the diameter of the gold particles is 1±0.1 μm. The theoretical full width at half maximum of the SPP virtual probe is 261 nm (~0.245 λ 0 ). Full size image Sequential snapshots extracted from charge-coupled device (CCD) video ( Fig. 2a,b , see Supplementary Movie 1 ) reveal that the plasmonic virtual probe is able to attract nearby particles as soon as the SPP field encounters the particle. Particles can also be dragged by the virtual probe over large distances (>5 μm from the centre), indicating that the force is sufficiently strong for any physical manipulation. More trapping experiments for dielectric and metallic particles in the diameter range 0.5–2.2 μm (see Supplementary Fig. S2 and Supplementary Movie 1 ) demonstrate that plasmonic tweezers can trap both dielectric and metallic particles, with an effective large size range from nanometre to micrometre. 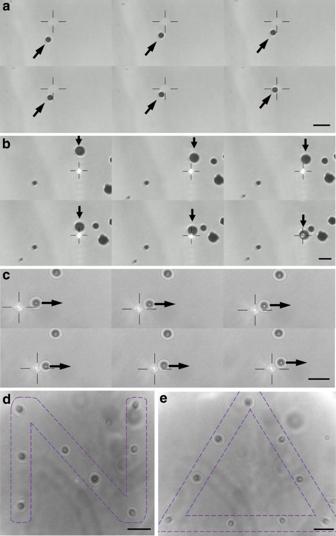Figure 2: Comparison of plasmonic and optical tweezers experiments. (a) Successive images of gold particles (diameter of 1±0.1 μm) trapped by the focused plasmonic tweezers recorded using a CCD camera. The image sequence is from top left to bottom right with a time interval between images of 1/5s. The black arrow indicates the direction of particle motion, and the black cross indicates the position of the plasmonic virtual probe. (b) Successive images of gold particles (diameter of 2.2±0.1 μm) trapped by the focused plasmonic tweezers with a time interval of 1/2s. (c) Successive images of gold particles (diameter of 1±0.1 μm) pushed by optical tweezers with a time interval of 21/15s. The incident beam and experimental configuration is the same as for (a) but without the metal film on the chamber surface. The light spot indicated by the black cross is moving from left to right, pushing the particle as indicated by a black arrow. (d,e) Patterns of the letter ‘N’ and triangle ‘▵’ constructed by gold particles (diameter of 1±0.1 μm) in the focused plasmonic tweezers. The length of all scale bars (black line in lower right corner) is 3 μm. Figure 2: Comparison of plasmonic and optical tweezers experiments. ( a ) Successive images of gold particles (diameter of 1±0.1 μm) trapped by the focused plasmonic tweezers recorded using a CCD camera. The image sequence is from top left to bottom right with a time interval between images of 1/5s. The black arrow indicates the direction of particle motion, and the black cross indicates the position of the plasmonic virtual probe. ( b ) Successive images of gold particles (diameter of 2.2±0.1 μm) trapped by the focused plasmonic tweezers with a time interval of 1/2s. ( c ) Successive images of gold particles (diameter of 1±0.1 μm) pushed by optical tweezers with a time interval of 21/15s. The incident beam and experimental configuration is the same as for ( a ) but without the metal film on the chamber surface. The light spot indicated by the black cross is moving from left to right, pushing the particle as indicated by a black arrow. ( d , e ) Patterns of the letter ‘N’ and triangle ‘ ▵ ’ constructed by gold particles (diameter of 1±0.1 μm) in the focused plasmonic tweezers. The length of all scale bars (black line in lower right corner) is 3 μm. Full size image Opposing behaviour is observed when the metallic-coated glass plate is replaced by a bare glass plate ( Fig. 2c ; see also Supplementary Movie 2 ). Particles are seen being pushed away when the focused optical beam falls on the plate. Plasmonic manipulation of metallic particles The polarization rotator (PR) system ( Fig. 1b ) is able to switch between radial polarization and azimuthal polarization; as the SPPs are sensitive to the polarization of the incident light, we can therefore control the presence of the virtual probe. A designed shape can be realized by trapping gold particles to certain locations one by one. In the experiment, we used a glycerine–water solution (volume ratio 1:4) to reduce the Brownian motions of gold particles in the chamber. As seen in Fig. 2d,e , about 10 Au particles were manipulated dynamically to pattern the letter ‘N’ and a triangle ‘ ▵ ’. Our method thus has potential for application in micronano fabrication, as well as enhancing Raman signals in specific locations. Calculation of forces on particles in both types of tweezers To understand the experimental observations, we performed numerical analysis, based on an FDTD calculation and MST method, of the forces involved in these two experimental configurations (see Methods for the analytical procedure). The resultant electrical field distributions and Poynting vectors, total forces, gradient forces and scattering forces exerted on the particle are presented for comparison in Fig. 3 . 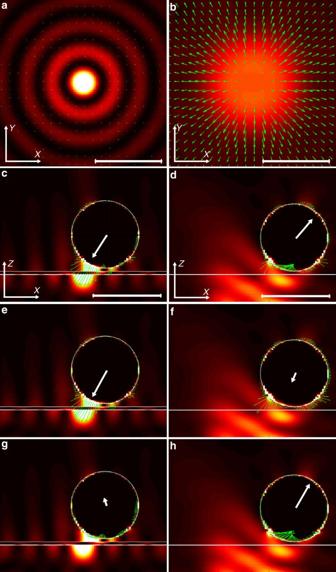Figure 3: Comparison of forces in plasmonic and optical tweezers. Distribution of electric field intensity (background) and Poynting vector (green arrows) in the horizontalx-yplane of (a) the focused plasmonic tweezers and (b) the focused optical tweezers, where thex-yplane is 50 nm above the gold–water interface in (a) and the glass–water interface in (b), respectively. (c), (e) and (g) show the total force, gradient force and scattering force, respectively (green arrows), distributed on a gold particle (diameter of 1 μm) in the verticalx-zplane for the plasmonic tweezers. The background is the electric field intensity, while the white lines indicate the spherical particle and gold film. The particle with a diameter of 1 μm is 50 nm above the gold surface and 300 nm away from the SPP peak at the horizontal centre. (d), (f) and (h) show similar cases to (c), (e) and (g), respectively, except for the optical tweezers without metal film and the particle is 600 nm away from the horizontal centre. The white arrow starting from the centre of the sphere in (c–h) denotes the resultant force on the particle. The length of all scale bars (white line in lower right corner) is 1 μm. Other simulation parameters are as follows: the incident wavelength isλ0=1,064 nm, the thickness of the gold film is 45 nm, the refractive index of the glass substrate is 1.515. Figure 3: Comparison of forces in plasmonic and optical tweezers. Distribution of electric field intensity (background) and Poynting vector (green arrows) in the horizontal x-y plane of ( a ) the focused plasmonic tweezers and ( b ) the focused optical tweezers, where the x-y plane is 50 nm above the gold–water interface in ( a ) and the glass–water interface in ( b ), respectively. ( c ), ( e ) and ( g ) show the total force, gradient force and scattering force, respectively (green arrows), distributed on a gold particle (diameter of 1 μm) in the vertical x-z plane for the plasmonic tweezers. The background is the electric field intensity, while the white lines indicate the spherical particle and gold film. The particle with a diameter of 1 μm is 50 nm above the gold surface and 300 nm away from the SPP peak at the horizontal centre. ( d ), ( f ) and ( h ) show similar cases to ( c ), ( e ) and ( g ), respectively, except for the optical tweezers without metal film and the particle is 600 nm away from the horizontal centre. The white arrow starting from the centre of the sphere in ( c – h ) denotes the resultant force on the particle. The length of all scale bars (white line in lower right corner) is 1 μm. Other simulation parameters are as follows: the incident wavelength is λ 0 =1,064 nm, the thickness of the gold film is 45 nm, the refractive index of the glass substrate is 1.515. Full size image In Fig. 3a,b , typical field patterns are shown for the focused plasmonic and optical tweezers corresponding to the horizontal plane ( x – y plane) above the gold–water and glass–water interfaces, respectively. Note that the central peak is much tighter and much stronger for the SPP field than for the optical field. However, the Poynting vectors (marked by green arrows) for the SPP field almost disappear compared with that for the optical field, which imply physically that the power flux for the plasmonic tweezers is much lower than that for the optical case. These differences provide clues to understanding the pull instead of push exerted by the plasmonic tweezers. The total force, composed of gradient and scattering forces ( Fig. 3c,d ), mainly indicates left and right horizontal directions, respectively, concordant with the experiments. However, further decomposition reveals an intriguing fact. As displayed in Fig. 3e,f , both gradient forces tend to attract particles towards the centre, although the plasmonic tweezers produced a much stronger force. In Fig. 3g,h , the scattering force for the optical tweezers opposes the gradient force, whereas the scattering force for the plasmonic tweezers in contrast augments the gradient force in the horizontal direction. Force analysis from particle movement for plasmonic tweezers We also studied the total force exerted on the particle by directly analysing the particle motion in the experiments of plasmonic tweezers (see Methods for the analytical procedure). As plotted in Fig. 4a , the black dot represents these experimental outcome data points. We can see that they follow the same trend as the numerical results when close to the virtual probe. In Fig. 4b , we also plot the one-dimensional distribution of forces along the vertical direction ( F z ), which is found to be different from the horizontal forces ( F x ): the former increase exponentially in magnitude all the way when close to the gold film, while the latter reach a maximum and then decrease in magnitude when close to the SPP virtual probe centre. For F x , both force components (gradient and scattering) follow the same trend, while they show opposite behaviour in F z . 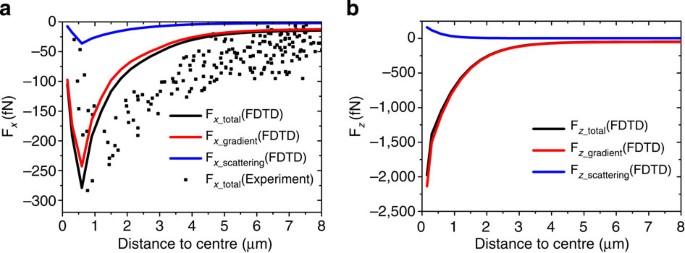Figure 4: Horizontal and vertical forces versus particle positions in plasmonic tweezers. (a) Horizontal force (Fx) and (b) vertical force (Fz) exerted on a metallic particle in focused plasmonic tweezers at different particle positions. Abscissa represents the distance between the particle centre and the central peak of the SPP virtual probe. All solid curves are theoretical results based on FDTD and MST calculations; the black dots represent experimental data. For all theoretical results, particle diameters are 1 μm, and for all experimental results only particles of diameter 1±0.1 μm were chosen. Figure 4: Horizontal and vertical forces versus particle positions in plasmonic tweezers. ( a ) Horizontal force ( F x ) and ( b ) vertical force ( F z ) exerted on a metallic particle in focused plasmonic tweezers at different particle positions. Abscissa represents the distance between the particle centre and the central peak of the SPP virtual probe. All solid curves are theoretical results based on FDTD and MST calculations; the black dots represent experimental data. For all theoretical results, particle diameters are 1 μm, and for all experimental results only particles of diameter 1±0.1 μm were chosen. Full size image For metallic particles, the attractive gradient force is essentially the Coulomb force that depends on the local electric field and the charge density induced in the particle. The pushing scattering force meanwhile is the Laplace force related to the local magnetic field [18] . Thus, the gradient force can be enhanced by a stronger and sharper electric field and always points to the peak of the field, whereas the scattering force is determined by the light propagation as well as the power flux. In our plasmonic tweezers, the successful trapping of metallic particles is, as stated earlier, due to an SPP-enhanced gradient force accompanied by a scattering force in the horizontal direction ( Fig. 3e,g ). The key to the unusual contribution of the force is the highly focused SPP virtual probe field, whose full width at half maximum of focus is sized in deep subwavelength (~0.245 λ 0 ) because the plasmonic wave is an evanescent wave beyond the diffraction limit. Compared with the diffraction-limited focusing of a Gaussian beam in ordinary optical tweezers, the sharper focusing of the plasmonic wave produces stronger gradient forces. Further, the scattering force in our plasmonic-trapping system aligns with the gradient force, and therefore helps trapping. Thus, even if a Gaussian beam can be focused up to the size of the virtual probe, it is still very hard to trap the mesoscopic/Mie size metal particle, because as the focus size decreases, the repulsive scattering force of the Gaussian beam strengthens more rapidly than the gradient force at the focus region, and therefore disrupts the trapping. In plasmonic tweezers, the generating process of the virtual probe is similar to that described in refs 23 , 24 . First, the SPPs are excited by a focused PR beam at a typical surface plasmon resonance (SPR) angle, and then act as secondary circular sources on the metal film propagating inward to the centre, and finally form sharp and strong plasmonic virtual probes after constructive interference. In this process, the scattering force derives from the pushing as excited SPP propagate inward towards the central peak; the direction of push is hence in the same direction as the attractive gradient force. However, the scattering force is weaker than the gradient force because after interference the final focused SPP field approximates a standing wave pattern and thus produces a low power flux (as evidenced by the Poynting vectors in Fig. 3a ). In the region of SPP field, metal particles are first attracted by the side lobes around the virtual probe, and then dragged by the gradient force to the centre and finally trapped. The dominant gradient force originates from the greatly enhanced coupling between the SPP field and the metallic particle (as seen in Fig. 3e by the high-field intensity at the lower left surface of the particle). When the particle approaches the SPP virtual probe centre, the gradient force first reaches a maximum because of the increasing field intensity, and then decreases in magnitude at the centre as a result of force equilibrium in the horizontal direction ( Fig. 4a ), which enables a potential well to form in which to confine the particle. The dominant role of the gradient force is also reflected in Fig. 4b because the vertical force correlates strongly with coupling strength. In contrast, for the optical tweezers without metal film, the optical focus is not as sharp as the plasmonic virtual probe; the coupling between optical focus and metallic particle is weak ( Fig. 3f ), while the power flux from centre to outer is strong ( Fig. 3b ). Thus, with the scattering force being greater than the gradient force, metallic particles are pushed away from the focus. For similar reasons, in the unfocused SPP field, the metallic particles are also pushed away by the stronger scattering force [19] . Besides optical gradient and scattering forces, it was reported that the heating effects, including thermophoresis and convection, play a complicated role in plasmonic trapping systems [26] , [27] , [28] , [29] , [30] , [31] . Thermophoresis can generate forces either in the direction of heat gradient or in the opposite direction [31] , while the convection could help trapping by circulating fluid around, to draw particles to the hot region [26] . In our plasmonic trapping system, because only a very small amount of incident light could couple to SPP and contribute to the heating effect, and the heat is rapidly conducted to the whole-gold film because of the high thermal conductivity, the final temperature increase in the plasmonic trapping system is maintained in the order of several degrees Kelvin (see Supplementary Fig. S3a ). This temperature increase creates a convection force by circulating fluid (see Supplementary Fig. S3b ) to further strengthen the trapping force along the horizontal dimension. Hence, in Fig. 4a the experimental force is slightly stronger than the theoretical expectation of the optical force in some regions. In conclusion, our research revealed an unusual feature between the gradient and scattering forces in our focused plasmonic tweezers, enabling stable traps of metallic particles, especially in the mesoscopic/Mie size range. In contrast to the push incurred by particles in optical tweezers due to the stronger scattering force, the SPP-enhanced gradient force in plasmonic tweezers dominates. Augmented by a like-directed scattering force, metallic particles are therefore attracted towards the central peak of the highly focused SPP field. Theoretical results obtained by 3D FDTD simulations agree well with the experimental data, disclosing that the key to the successful trapping of particles in plasmonic tweezers is the highly focused SPP field. Besides mesoscopic/Mie metallic particles, the plasmonic tweezers are also capable of trapping dielectric particles and Rayleigh metallic particles, which although easier, is beyond the scope of this paper. Thus, such plasmonic tweezers could be employed for trapping and manipulating various metallic objects from nanometre to micrometre scales. Moreover, because of the enhancement from coupling between SPPs and localized surface plasmons of the metallic particles, the plasmonic tweezers have great potential in surface-enhanced Raman scattering [32] , [33] , [34] and other applications. We believe that this work not only provides a different way of trapping and manipulating metallic particles but also delivers an important contribution towards a comprehensive understanding and optimization of trapping forces produced by SPP-enhanced evanescent fields. Excitation of SPP virtual probe in plasmonic tweezers The detailed experimental set-up for excitation of SPP virtual probe is shown in Fig. 1b . The incident beam (100 mW, 1,064 nm) is first circularly polarized by passing through a polarizer and a λ /4 waveplate, and then azimuthally polarized using a spiral phase plate and an azimuthal analyser. It is finally RP by a PR, which consists of two half-wave plates, and which can also alternate the polarization state of the beam between azimuthal and radial polarization by turning one plate by 45°. A telescope system composed of a spiral phase plate between two lenses collimates and broadens the generated RP beam illuminating the back aperture of the objective lens. The gap between the objective lens and the glass substrate is filled with index-matching oil ( n =1.515). The samples are gold particles diffused in water and injected into an in-house-fabricated well. A white-light source illuminates the samples from the top for direct imaging using a CCD camera and observation of the gold particles. As the numerical aperture of the objective lens is 1.49, the maximum incident angle on the gold film (thickness of 45 nm) extends to 79.6°, satisfying both the requirements of SPP excitation and clear observation of particles via CCD. As the focused RP beam has a transverse magnetic polarization with respect to the metal film, SPPs can be excited on a metal film at SPR angle (~44.5°), resulting in a near-zero reflection. To confirm the excitation of SPPs in our plasmonic tweezers, we recorded the image of reflected light at the back focal plane of the objective lens using a CCD camera (see Supplementary Fig. S1a ). The sharp dark ring corresponding to near-zero reflection at the SPR angle verifies that the incident RP beam has efficiently excited a ring-shaped SPP, which couples to the metal film to form the SPP virtual probe at the centre. To show the characteristics of the plasmonic virtual probe, we present both experimental measurement and FDTD simulation of near-field intensity distribution of the virtual probe on a thin gold film (see Supplementary Fig. S1b–d ). When the gold film is located before the focal plane of the objective lens, the excited SPP acts as a secondary circular source propagating towards the centre. As a result, a sharp peak (virtual probe) of ultra-high intensity is formed at the centre by SPP constructive superposition, which can serve as a highly concentrated source to trap metallic particles (as shown in Fig. 1a ), similar to hot spots in the metallic bowtie-trapping structures [22] . Theoretical calculation of total electromagnetic force To obtain further insight into the trapping and pushing of gold particles as employed in the experiments, we calculated in a 3D FDTD [35] simulation the electric field distributed around the particle, and further applied the MST method to obtain the total electromagnetic force exerted on the particle, for both types of tweezers. All simulation parameters were chosen to match experimental conditions. The grid size is non-uniform ranging from 5 nm near material interfaces to 25 nm further from these boundaries. The focusing field after a high numerical aperture lens is used as the input source in the FDTD simulation. Although we do not know the actual vertical distance d between the bottom of the gold particle and the top of the metal film, we chose d =50 nm in all simulations in accord with the Debye length, which is a typical length for electrostatic interactions commonly used in similar computations [19] . For the MST method, denoting the three force components by F x , F y and F z , the time-average force F can be written as [36] : where ε and μ are the relative permittivity and relative permeability of the medium around the particle, and n is the unit normal perpendicular to the integral area d s . The electric and magnetic field components required in the MST method are obtained directly from the FDTD simulation data. The detailed derivation of equation (1) is given in Supplementary Note 1 . Here we only consider the two-dimensional trapping in the x–y plane on the metal surface. Therefore, trapping or pushing only depends on horizontal forces F x and F y . Further, owing to the cylindrical symmetry of incident light, only F x needs to be considered in describing trapping if we choose y =0 for the position of the particle. Theoretical calculation of gradient and scattering forces The MST method only gives the total electromagnetic force exerted on the particle. To understand the different mechanisms underlying the two types of tweezers, we need to further separate the total electromagnetic force into gradient and scattering forces. For Rayleigh metallic particles, it is easy to calculate these two forces using the dipole approximation model [9] . However, it is not suitable for mesoscopic and Mie metallic particles. Here we develop an alternative method to calculate these forces for mesoscopic/Mie metallic particles based on the MST method. According to classical electromagnetic theory, the total electromagnetic force (Lorentz force) is with the gradient force associated with the electrical field and the scattering force associated with magnetic field are [18] Thus, we can calculate the gradient and scattering forces by integrating the tensor and , which are given in Note here all electric and magnetic field components in the x , y and z directions are obtained from FDTD simulation data. A detailed derivation of equations (7) and (8) is described in Supplementary Note 2 . In contrast to the well-known optical gradient force that basically depends on the gradient of the intensity [9] , here the gradient force for a large metal particle is more complicated and determined by both amplitude and phase of the electric field components on the particle surface. Total force calculation from experimental particle movements To verify the theoretical results, we calculated the total force from particle motion in the horizontal plane of the experimental set-up. This is based on , where is the acceleration of the particle and F drag is the drag on the particle in solution. Here, however, we consider the acceleration term simply for a more complete description. Indeed, the acceleration term is usually several orders of magnitude smaller than the drag term. The velocity v and acceleration for the particle dynamics can be extracted from the videos captured using the CCD camera. The drag exerted on particles in solution can be calculated from F drag = μ v with drag coefficient μ =6 πηa , where η is the dynamic viscosity of water and a particle radius. Note that the drag coefficient increases when the particle is approaching the surface (Faxen’s law) [37] and the viscosity η decreases with increasing temperature [29] . Thus, we modify the drag coefficient according to the vertical distance of the particle ( d =50 nm, same as the FDTD simulation) and the temperature increase near the metal surface (see Supplementary Fig. S3a ). The calculated experimental trapping force is shown in Fig. 4a , which follows the same trend as the FDTD results. The slight difference between experimental and FDTD results in Fig. 4a might be due to thermal convection forces (see Supplementary Fig. S3b ) and experimental deviations. How to cite this article: Min, C. et al. Focused plasmonic trapping of metallic particles. Nat. Commun. 4:2891 doi: 10.1038/ncomms3891 (2013).